Microgels on-demand Three-dimensional (3D) hydrogel structures are finding use in fundamental studies of self-assembly, rheology, and 3D cell culture. Most techniques for 3D hydrogel formation are ‘single pot’, in which gels are not addressable after formation. For many applications, it would be useful to be able to form arrays of gels bearing mixtures of constituents and/or formed from composites of different gel materials. Here, in response to this challenge, we introduce a digital microfluidic method for ‘on-demand’ formation of arrays of microgels bearing arbitrary contents and shapes. On formation of the gels, each microgel is individually addressable for reagent delivery and analysis. We demonstrate the utility of the method for 3D cell culture and higher-order tissue formation by implementing the first sub-microlitre recapitulation of 3D kidney epithelialization. We anticipate this platform will enable new research that can exploit the flexible nature of this technique for forming and addressing arrays of hydrogels with unique geometries and contents. Precision polymer gels with sub-mm dimensions (or ‘microgels’) are used in tissue engineering [1] , stimulus-responsive materials [2] , sample preparation for mass spectrometry [3] , bar coding for chemistry [4] and flexible photonic crystals [5] . A number of strategies relying on microchannels have been developed for microgel formation relying on continuous flows [6] , [7] , [8] and two-phase systems consisting of droplets in a carrier fluid. [9] , [10] . Surface tension effects have restricted two-phase flow systems to the formation of monodisperse spherical, disc or rod-shaped solids produced by either photo-initiation or thermal cross-linking at a T-junction or by flow-focusing [11] , [12] , [13] . After formation, phase separation requires compatible chemistries to isolate microgels from the immiscible phase. Recently, single-phase stop-flow lithography was introduced, which enables the formation of microgels in diverse geometries [14] , [15] . This is important, as arbitrarily shaped microgels are useful for providing novel insights on the relationship between the microenvironment and cell fate and behaviour [16] . Stop-flow lithography is useful for UV-initiated cross-linked polymers; however, the method is not compatible with chemically and thermally cross-linked polymer systems, which are widely used for three-dimensional (3D) cell culture. Micromoulding techniques [17] , [18] , in which hydrogels are cast and released from silicone moulds, are not subject to these limitations (allowing for chemically and thermally cross-linked gels), but the types of shapes that are formed must be pre-defined. Most importantly, all of the systems described above are ‘single pot’ methods, such that all gels have the same constituents, and they are not individually addressable after formation. Digital microfluidic (DMF) liquid handling ( Fig. 1 ) is an emerging alternative to the paradigm of enclosed microchannels [19] . This technology facilitates electrostatic manipulation of discrete nano- and micro-litre droplets across open-electrode arrays providing the advantages of single-sample addressability, automation and parallelization. Variations of this platform have been demonstrated for a broad range of applications, including proteomics [20] , [21] , cell culture and analysis [22] , [23] , [24] , immunoassays [25] , [26] , chemical synthesis [27] , [28] and on-chip lasing [29] . Recently, the unique geometry of DMF has been exploited for handling and addressing of 3D solids, such as paper discs for genetic screening [30] , [31] , polymer monoliths for sample extractions [32] and agarose discs for scaffolding applications [20] , [33] . 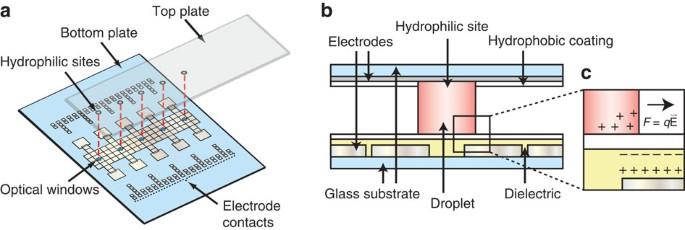Figure 1: DMF device geometry. (a) Exploded view of device, comprising a bottom plate with patterned electrodes and a top plate bearing patterned hydrophilic sites. (b) Side-view of device, not to scale. (c) Schematic depicting principle of device operation. Figure 1: DMF device geometry. ( a ) Exploded view of device, comprising a bottom plate with patterned electrodes and a top plate bearing patterned hydrophilic sites. ( b ) Side-view of device, not to scale. ( c ) Schematic depicting principle of device operation. Full size image Motivated by the challenges of microgel formation and addressability, we sought to exploit recent developments in reagent dispensing and the handling of solids on DMF devices for microgel formation. Here we report a DMF method for: (1) on-demand microgel formation, (2) flexible microgel geometries, (3) single microgel addressability and (4) compatibility with UV, chemical or thermally cross-linked polymer systems. We call the new technique microgels on-demand, defining ‘on-demand’ as the capacity to generate a 3D gel structure containing any arbitrary combination of constituents in situ . We demonstrate that the new method is a useful new tool for culturing and analysing meso-scale 3D cell constructs that are difficult to work with using conventional methods. We propose that microgels on-demand represents a useful new tool for 3D cell culture and other hydrogel-based techniques [34] . Microgels on-demand To form microgels on-demand, droplets of sol-phase hydrogel are manipulated across hydrophilic sites on a DMF device to form sub-droplets by line pinning ( Fig. 2 ). This technique has been used previously for non-gelling fluids (known in DMF as ‘passive dispensing’ [22] and in non-DMF methods as ‘surface energy traps’ [35] ), but this is the first application to exploit this technique for hydrogels. Sub-droplets of sol-phase hydrogel materials deposited onto hydrophilic sites can be cross-linked to form pillar-shaped microgels. This process is highly reproducible, with volumetric precisions ranging from 0.3% to 8.1% ( Supplementary Fig. 1 ). 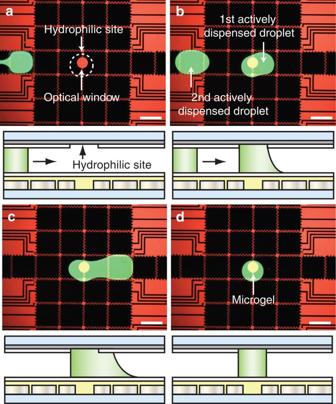Figure 2: Microgels on-demand. Frames from a movie (top) and side-view schematic (bottom) depicting a sol-state hydrogel droplet containing a fluorescent dye being dispensed from a reservoir (a) and then driven to a patterned hydrophilic site. A second droplet is then dispensed (b) and passed across the hydrophilic site (c), forming a sub-droplet in the shape of the site (d). On cross-linking, each droplet forms a solid microgel. Scale bars, 2 mm. Figure 2: Microgels on-demand. Frames from a movie (top) and side-view schematic (bottom) depicting a sol-state hydrogel droplet containing a fluorescent dye being dispensed from a reservoir ( a ) and then driven to a patterned hydrophilic site. A second droplet is then dispensed ( b ) and passed across the hydrophilic site ( c ), forming a sub-droplet in the shape of the site ( d ). On cross-linking, each droplet forms a solid microgel. Scale bars, 2 mm. Full size image Three thermally cross-linked hydrogels were used here: Geltrex (a reconstituted basement membrane complex of extracellular matrix (ECM) proteins [36] that remains in sol phase at temperatures below 4 °C), Type I collagen (an ECM protein that cross-links at neutral pH and 37 °C), and agarose (a gel that remains in sol phase at temperatures above 42 °C). Agarose microgels formed in this manner can be evaluated off-chip by environmental scanning electron microscopy ( Fig. 3a,b ), revealing that they possess the honeycomb structure typical of agarose microgels formed by other means [37] . UV and chemical cross-linking methods were also implemented to form polyacrylamide and alginate hydrogels, respectively ( Supplementary Fig. 2 ). We propose that similar methods should be applicable to a wide range of hydrogel materials. 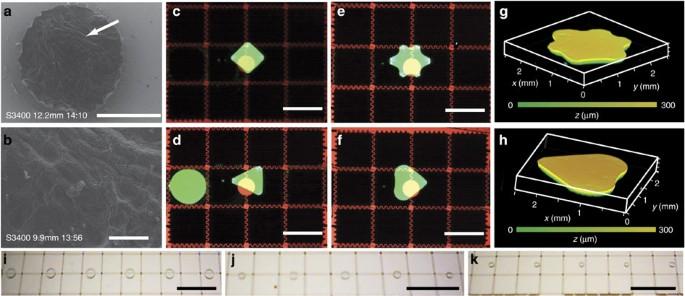Figure 3: Sizes and geometries of microgels. Environmental scanning electron microscopy images (a,b) of agarose (5% w/v) microgels formed and cross-linked on device. Scale bars, 1 mm and 100 μm, respectively. Various geometries can be generated and visualized with epifluorescent stereomicroscopy (c–f) or confocal microscopy (g,h). Scale bars, 1 mm. Geltrex microgels were formed with diameters of 1,000 μm (i), 750 μm (j), 500 μm (k). With heights of 75 μm, these microgels possess volumes of 60, 33, and 14 nl, respectively. Scale bars, 5 mm. Figure 3: Sizes and geometries of microgels. Environmental scanning electron microscopy images ( a , b ) of agarose (5% w/v) microgels formed and cross-linked on device. Scale bars, 1 mm and 100 μm, respectively. Various geometries can be generated and visualized with epifluorescent stereomicroscopy ( c – f ) or confocal microscopy ( g , h ). Scale bars, 1 mm. Geltrex microgels were formed with diameters of 1,000 μm ( i ), 750 μm ( j ), 500 μm ( k ). With heights of 75 μm, these microgels possess volumes of 60, 33, and 14 nl, respectively. Scale bars, 5 mm. Full size image The shapes of microgels formed on demand can be tuned simply by altering the shape of the hydrophilic sites for passive dispensing. For example, star-, heart- triangle- and diamond-shaped microgels were readily formed using the microgel on-demand technique ( Fig. 3c–f and Supplementary Movie 1 ). These non-cylindrical shapes are found to be conformal through the vertical axis by confocal microscopy ( Fig. 3g,h ). Interestingly, microgels with different heights can also be generated by using asymmetric inter-plate spacing; for example, Supplementary Movie 2 depicts the formation of microgels on a device with a 75-μm spacer on one side and a 300-μm spacer on the other side. The microgels used here were routinely formed with dimensions ranging from 500 μm to 2,000 μm diameter, and 75 μm to 225 μm height ( Fig. 3i–k ), which spans a microgel volume range of 14–700 nl. In the future, we propose that additional microgel sizes (larger or smaller) might be compatible with devices with different electrode and hydrophilic spot sizes. Addressable reagent delivery and composite microgels A key benefit of DMF liquid handling is the independent addressability of electrodes and thereby individual droplets. This feature allows for the targeted delivery of reagents, an important attribute for maintaining hydration, as well as for maintaining cell viability in 3D tissue culture. As shown in Supplementary Fig. 3 , droplets of reagents can be individually delivered to (and removed from) microgels by applying an appropriate sequence of driving potentials. This dispensing mechanism is reproducible and precise, ensuring that each passage delivers equal amounts of fresh reagent with volumetric precision varying from 0.29 to 3.29%. To examine diffusion into microgels generated on-demand, we used fluorescein (0.3 kDa), 4-kDa and 40-kDa FITC-dextrans as surrogates for the small molecules, growth factors and cytokines often used in cell culture and stimulation [38] . Specifically, droplets containing these tracers were delivered to Geltrex microgels formed on-demand and diffusion was tracked by fluorescence imaging. As shown in Fig. 4a–d , on delivery of a droplet, a film of tracer forms around the microgel and diffuses toward the centre. For comparison, diffusion was modelled numerically, which was found to be consistent with the experimental results ( Fig. 4e ). The three tracers had apparent diffusion coefficients ( D a ) in Geltrex of D a =10 × 10 −10 m 2 s −1 (fluorescein), 7.2 × 10 −11 m 2 s −1 (4-kDa FITC-dextran) and 3.1 × 10 −11 m 2 s −1 (40-kDa FITC-dextran), respectively ( Fig. 4f ). Further, the experimental values are consistent with the diffusion coefficients, D , reported in the literature for similar (but not identical) systems: fluorescein in water [39] ( D =4.9 × 10 −10 m 2 s −1 ) and Matrigel [40] ( D =4.2 × 10 −10 m 2 s −1 ), 8-kDa FITC-dextran in agarose [41] ( D =8 × 10 −11 m 2 s −1 ), 20-kDa FITC-dextran in water [42] ( D =8 × 10 −11 m 2 s −1 ) and agarose [38] ( D =4.2 × 10 −11 m 2 s −1 ). 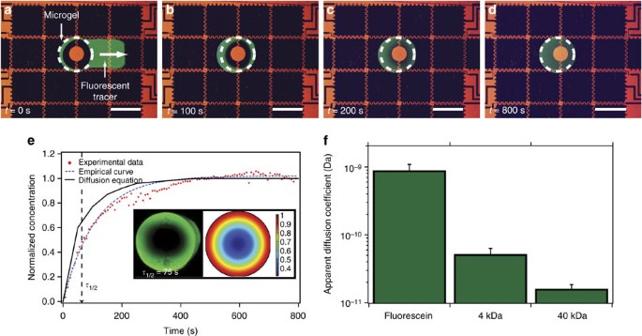Figure 4: Reagent exchange in microgels. (a-d) Frames from a movie depicting a droplet of fluorescein being driven across a (transparent) microgel and subsequent diffusion of fluorescein into the microgel. Scale bars, 2 mm. (e) Experimental (red dots), empirical fit (dashed blue line) and simulation (solid black line) of diffusion profiles for fluorescein into Geltrex microgels. The inset shows a fluoresecent image (left) and heat-map simulation of concentration (right) of fluorescein at the half-saturation point (τ1/2). (f) Apparent diffusion (Da) coefficients measured for fluorescein, 4 kDa FITC-dextran and 40 kDa FITC-Dextran into Geltrex. Error bars indicate 1 s.d. Figure 4: Reagent exchange in microgels. ( a - d ) Frames from a movie depicting a droplet of fluorescein being driven across a (transparent) microgel and subsequent diffusion of fluorescein into the microgel. Scale bars, 2 mm. ( e ) Experimental (red dots), empirical fit (dashed blue line) and simulation (solid black line) of diffusion profiles for fluorescein into Geltrex microgels. The inset shows a fluoresecent image (left) and heat-map simulation of concentration (right) of fluorescein at the half-saturation point ( τ 1/2 ). ( f ) Apparent diffusion ( D a ) coefficients measured for fluorescein, 4 kDa FITC-dextran and 40 kDa FITC-Dextran into Geltrex. Error bars indicate 1 s.d. Full size image Microgels can be generated on-demand in the form of arrays—for example, a 32-gel array is shown in Fig. 5a , and the individual addressability of the method allows the user to tailor the contents of each microgel in the array. This capacity is highlighted in Fig. 5b , which features an array of microgels containing mixtures of red, yellow and green tracers. The array was generated combinatorially on-device from three-stock sol-phase solutions (each containing only one colour of tracer) through a series of droplet merging, mixing and splitting steps. Finally, the individual addressability of the technique allows for the formation of composite microgels. As shown in Fig. 5c–e , initial gels can be formed from either Geltrex or agarose, followed by the generation of a secondary hydrogel structure enveloping the initial structure. 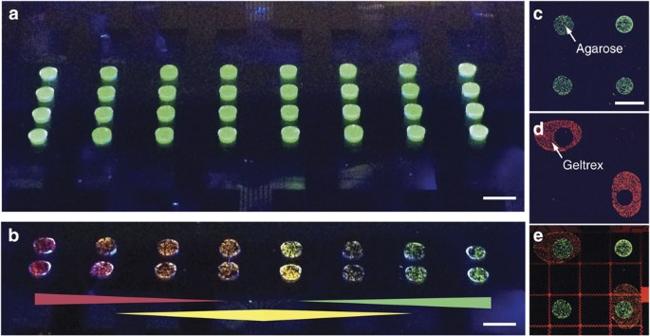Figure 5: Microgel arrays and composites. (a) A 32-plex array of microgels was formed from Geltrex supplemented with fluorescein for visualization. (b) A combinatorial array of Geltrex microgels was formed on device containing mixtures of red, yellow and/or green microspheres. Gradient bars indicate the per cent compositions of each respective microsphere, from 100% red at the left and 100% green at the right. (c–e) Composite microgels containing fluorescent microspheres were formed with inner agarose (with green microspheres) and outer Geltrex (with red microspheres) layers (c, green filter;d, red filter;e, composite image). Scale bars, 2 mm. Figure 5: Microgel arrays and composites. ( a ) A 32-plex array of microgels was formed from Geltrex supplemented with fluorescein for visualization. ( b ) A combinatorial array of Geltrex microgels was formed on device containing mixtures of red, yellow and/or green microspheres. Gradient bars indicate the per cent compositions of each respective microsphere, from 100% red at the left and 100% green at the right. ( c – e ) Composite microgels containing fluorescent microspheres were formed with inner agarose (with green microspheres) and outer Geltrex (with red microspheres) layers ( c , green filter; d , red filter; e , composite image). Scale bars, 2 mm. Full size image Microgel kidney epithelialization With the ability to form microgels on-demand by DMF and to address them independently for reagent exchange, we tested this system for 3D cell culture using the well-characterized model of kidney epithelialization [34] , [43] , [44] . Madin Darby canine kidney (MDCK) cells were suspended in sol-phase Geltrex and this suspension was used to form microgels on-demand, as above ( Fig. 6a ). Cells cultured in microgels remained viable in excess of 5 days, with delivery of fresh media droplets at 24-h intervals. At 4 h after seeding in microgels, viability was ~100%; while at 24 h after seeding, viability was ~80%. The effects of electrostatic actuation on cell health were not explicitly evaluated here, but previous studies with 2D adherent or suspension cell culture have reported no or negligible effects on cell viability/morphology [24] , [45] or gene expression [46] when compared with non-actuated cells (as the electrical field drops across the insulating layer rather than droplets containing cells). As shown in Fig. 6b and Supplementary Fig. 4 , MDCK cells were found to be suspended within the hydrogel matrix with a slight bias to the bottom of the device, with no cells adhered to either top or bottom plates. 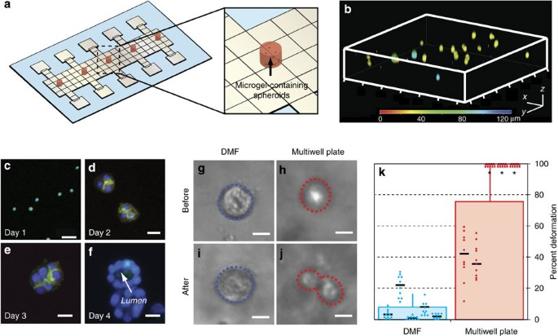Figure 6: Higher-order tissue formation and handling in microgels. (a) Cartoon depicting five microgels containing spheroids. The inset highlights one microgel containing spheroids. (b) Confocal microscopy image stack of MDCK cells in a Geltrex microgel demonstrates cell distribution throughout thezaxis. (c–f) Images depicting MDCK spheroid formation in a microgel over 4 days in culture. Cells were stained for actin with phalloidin (green) and nuclei with Hoechst (blue). On day 4, lumen formation was observed. (g–j) Representative bright-field images of day-4 MDCK spheroids pre- and post-exposure to five media exchanges by DMF or robotic pipetting. Scale bars, 20 μm. (k) Graph of spheroid deformation for five trials evaluating 10 spheroids each using robotic pipetting into a multiwell plate or DMF. The deformation value of each spheroid is indicated by a blue (DMF) or red (conventional reagent delivery) dot with black bars representing the mean deformation of each trial. Bar graphs show overall deformation averages across the five trials for each respective system. Error bars show 1 s.d. In three of the trials, identified by asterisks, the conventional method dislodged the hydrogels from the well, resulting in material failure. Figure 6: Higher-order tissue formation and handling in microgels. ( a ) Cartoon depicting five microgels containing spheroids. The inset highlights one microgel containing spheroids. ( b ) Confocal microscopy image stack of MDCK cells in a Geltrex microgel demonstrates cell distribution throughout the z axis. ( c – f ) Images depicting MDCK spheroid formation in a microgel over 4 days in culture. Cells were stained for actin with phalloidin (green) and nuclei with Hoechst (blue). On day 4, lumen formation was observed. ( g – j ) Representative bright-field images of day-4 MDCK spheroids pre- and post-exposure to five media exchanges by DMF or robotic pipetting. Scale bars, 20 μm. ( k ) Graph of spheroid deformation for five trials evaluating 10 spheroids each using robotic pipetting into a multiwell plate or DMF. The deformation value of each spheroid is indicated by a blue (DMF) or red (conventional reagent delivery) dot with black bars representing the mean deformation of each trial. Bar graphs show overall deformation averages across the five trials for each respective system. Error bars show 1 s.d. In three of the trials, identified by asterisks, the conventional method dislodged the hydrogels from the well, resulting in material failure. Full size image MDCKs form higher-order spheroid structures when cultured in collagen or matrigel matrices, making it possible to study epithelialization and primitive tissue formation in vitro [43] . To evaluate whether cells cultured in microgels on DMF can recapitulate this model, MDCKs were maintained on-device with daily media exchange for 1–4 days. On each day, the microgels were fixed, permeabilized and stained for actin and nuclei (all steps implemented by DMF as in Supplementary Fig. 3 , allowing for delivery of reagents in minutes). The inherent addressability makes this process straightforward, allowing for one gel to be stained and imaged on day 1 (while maintaining cell growth in the other gels), a second gel to be stained and imaged on day 2, and so on. The cells were observed to form multicellular clusters during the first 72 h, and a visible lumen after 96 h ( Fig. 6c–f ). Nuclei were distributed around the lumina with actin accumulation at the luminal edge, an indication of cellular polarization. Immunostaining for ZO-1 and E-cadherin provided further evidence of polarization of spheroids in microgels formed on-demand, with ZO-1 expressed along the luminal wall ( Supplementary Fig. 5 ). Further, the sizes of spheroids cultured within sub-microlitre microgels were similar to those grown in 96-well plates in 100-μl hydrogel aliquots ( Supplementary Fig. 6 ). Reagent exchange for cells grown in soft hydrogels is known to be problematic; in fact, in some such systems, cells are never fed with new media to avoid gel destruction, which limits the duration of experiments (P. Gilbert, University of Toronto, personal communication). To evaluate reagent exchange-induced damage in this system, we examined day-4 spheroids (cultured either in microgels on DMF devices or in wells on microtitre plates) by imaging before or after delivering and removing five aliquots of PBS. Deformation was determined by calculating the change in circularity of each spheroid’s 2D projection imaged by light microscopy ( Fig. 6g–j ). As shown in Fig. 6k , in five trials (evaluating 10 spheroids per trial), DMF handling of microgel-bearing spheroids resulted in a nearly tenfold reduction in deformation when compared with conventional fluid delivery to macro-scale hydrogels in multiwell plates: 7.6% for DMF and 75.9% for conventional methods. Of particular note are three trials in which conventional handling of the macro-scale hydrogels resulted in complete hydrogel displacement (quantified as 100% deformation), in which spheroids were disrupted to the extent that they could no longer be identified. Given the ability to recapitulate MDCK spheroid formation in microgels formed on-demand, we used the technique to implement a pilot screen to evaluate microenvironmental influences on spheroid characteristics. A panel of conditions was probed, including microgel content (Geltrex, Type I collagen, and mixtures of the two), microgel size (heights of 75 or 225 μm) and extracellular stimulation (incubation in exogenous hepatocyte growth factor, HGF, for 24 or 48 h). A total of 48 microgels were seeded on six devices and ~500 spheroids were imaged ( Fig. 7a,b ). Spheroids formed in microgels containing Type I collagen had significantly larger cross-sectional areas than those cultured in Geltrex: 1,450 and 810 μm 2 with 95% confidence intervals of 23% and 18%, respectively ( Fig. 7c ). In addition, spheroids formed in collagen were significantly more irregular in shape with mean roundness of 0.75 versus roundness of 0.82 for spheroids cultured in Geltrex ( Fig. 7d ). The effects of collagen were observed even when Geltrex was included in the matrix ( Supplementary Fig. 7 ). No significant changes in size or roundness were observed for microgels with reduced heights or in microgels exposed to HGF. 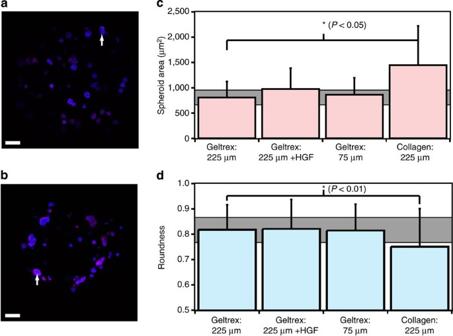Figure 7: Pilot screen for microenvironment effects on spheroid growth. Confocal images of spheroids formed in Geltrex (a) and Type I collagen (b) with cells stained for nuclei (blue) and actin (red). White arrows indicate representative spheroids; scale bars, 100 μm. Spheroids cultured in collagen microgels were larger (c) as measured by cross-sectional area, and more irregular (d) as measured by roundness. Exposure to HGF and reduction of inter-plate spacing (75 versus 225 μm) did not affect spheroid characteristics significantly. Error bars are+1 s.d., and shaded regions indicate 95% confidence intervals.P-values determined byt-tests. Figure 7: Pilot screen for microenvironment effects on spheroid growth. Confocal images of spheroids formed in Geltrex ( a ) and Type I collagen ( b ) with cells stained for nuclei (blue) and actin (red). White arrows indicate representative spheroids; scale bars, 100 μm. Spheroids cultured in collagen microgels were larger ( c ) as measured by cross-sectional area, and more irregular ( d ) as measured by roundness. Exposure to HGF and reduction of inter-plate spacing (75 versus 225 μm) did not affect spheroid characteristics significantly. Error bars are+1 s.d., and shaded regions indicate 95% confidence intervals. P -values determined by t -tests. Full size image Microgels on-demand is a DMF method for forming and using micron-dimension hydrogel structures. While DMF has been used for applications involving hydrogels [20] , [33] , the methods described previously are incapable of microgel formation and require extensive manual intervention (that is, gel structures are formed off-chip and then transferred one-by-one onto devices). In contrast, the new method reported here allows for the rapid and straightforward generation of arrays of microgels on-chip, where they are immediately ready to use for analysis. The new method reported here joins a list of several non-DMF techniques that are used to form microgels, including stop-flow lithography [14] , [15] , micromoulding [17] , [18] and gel-spotting [47] . The DMF technique has some advantages relative to the alternatives—for example, microgels on-demand: (a) is not limited to UV cross-linking (unlike stop-flow lithography), (b) forms microgels with individually tailored content in an array format for on-chip experiments (unlike stop-flow lithography and micromoulding) and (c) does not require robotics or moving parts (unlike gel spotting). But of course, the new technique also has some disadvantages: the sizes of the microgels described here are larger (500 μm versus <100 μm), and the throughput (hundreds per day versus more than tens of thousands per day) is lower relative to some of the alternate techniques. We propose that the different methods are complementary, and might be suitable for different applications. We chose 3D kidney epithelialization as a test case for the new method, because it is a widely studied model [34] , [43] , [44] of higher-order cell assembly (quite different from ‘spheroids’ that agglomerate in pre-formed targets or moulds [18] , [48] ). Until now, this system has never been tested in microgels—such structures have only been formed by pipetting into hydrogel-filled multiwell plates. Unfortunately, these conventional methods are tricky, and in fact, the simple act of delivering reagents to such structures is known to cause morphological damage [49] , particularly for cells grown in hydrogels with low viscoelastic storage modulus (~10 Pa for 50% Matrigel [50] , an ECM mixture similar to the Geltrex used here). We hypothesized that DMF, which has been previously reported to be useful for gentle handling of weakly adhered apoptotic cells [24] , might also be useful for non-disruptive reagent delivery to cell constructs grown in 3D microgels. The results in Fig. 6k support this hypothesis, indicating that the new technique is superior to conventional techniques for gentle handling of hydrogels, an important factor in terms of the cost benefit of 3D cell culture. Further, to probe the capabilities of the new technique for on-chip analysis, a pilot screen was devised to evaluate spheroid phenotype as a function of microgel geometry and content. The results ( Fig. 7 ) are consistent with previous reports [51] (generated in multiwell plates) indicating that Type I collagen gels permit branching/tubulogenesis in MDCK spheroids, whereas gels formed from ECM mixtures suppress these effects. We propose that the results presented here represent one example of vast experimental space that might be explored in the future using the new technique. For example, an array of microgels with different shapes might be formed to evaluate the relationship between the geometry of the environment and cell fate and behaviour [16] , [52] , or an array of microgels featuring different composites might be used to evaluate multi-scaffold chemistries for tissue-engineering applications [53] , [54] . Further, given the many uses [2] , [3] , [4] , [5] of hydrogels for applications outside of tissue engineering, we propose that microgels on-demand may represent a powerful new tool for chemistry, biology, physics, and beyond. Reagents Unless stated otherwise, general-use chemicals were from Sigma-Aldrich (Oakville, ON, Canada) or Fisher Scientific Canada (Ottawa, ON, Canada), antibodies, fluorescent dyes and cell media components were from Invitrogen/Life Technologies (Burlington, ON, Canada) and photolithography reagents were from Rohm and Haas (Marlborough, MA). Deionized (DI) water had a resistivity of 18 MΩ cm at 25 °C. DMF device fabrication DMF devices were fabricated using standard photolithography and metal etching, as detailed previously [22] . The bottom-plate device design featured an array of 2.2 × 2.2 mm chromium actuation electrodes and in certain cases included an array of 1-mm-diameter optical windows (that is, circular regions free from chromium) with 9 mm between each window. Each window straddled the interface between two actuation electrodes. DMF device top plates bearing hydrophilic sites were formed by performing a Teflon liftoff procedure on ITO-coated glass substrates as detailed previously [22] . The sites were 0.5–2 mm in diameter and were formed in arrays of 5, 8, 16 or 32 per substrate. The sites had circular, star, heart or diamond geometries, and the diameter for non-circular shapes was defined as the diameter of the smallest circle that would enclose the feature. DMF device assembly and operation The two plates were joined by 1–4 layers of double-sided tape (each layer ~75 μm), and aligned such that the edge of the top plate was adjacent to the outer edges of the reservoir electrodes on the bottom plate. Care was taken to align top and bottom plate features vertically (windows on the bottom plate and hydrophilic sites on the top plate). Before cell experiments, DMF top and bottom plates were sterilized in 70% ethanol for 10 min. Excess ethanol was shaken off and devices were permitted to air dry for 30 min within a biosafety cabinet. Devices were then assembled with an ITO-glass top plate and a chromium-glass bottom plate. An open-source, automated DMF actuation system called ‘DropBot’ (described in detail elsewhere [55] ) was used to program and manage the application of driving potentials of 120–140 V RMS generated by amplifying the sine wave output of a built-in function generator operating at 10 kHz. Reagents were loaded and dispensed, moved and merged as described previously [22] . In all DMF experiments, reagent solutions were supplemented with 0.02% Pluronics F68 except for sol-state Geltrex and collagen that were supplemented with 0.02% Pluronics F127 (ref. 56 ). Imaging during droplet manipulation was performed with a built-in webcam [55] . Thermally cross-linked microgel formation and addressing Devices bearing droplets were imaged with a CCD camera (Basler, Ahrensburg, Germany) mounted on a fluorescence-equipped stereomicroscope (Leica, Wetzlar, Germany). Geltrex was prepared by 1:1 dilution in DMEM supplemented with 10% FBS and 0.02% F127. The solution was maintained on ice until device loading. Low gelling temperature agarose microgels were prepared as 1–6% w/v solutions in DI water by microwaving the solution for 30 s before device loading. In some cases, sol-state hydrogel solutions were supplemented with 10 μM fluorescein or with a suspension of fluorescently labelled (green, yellow or red) 10-μm diameter microspheres. To form microgels, 5 μl of sol-state or precursor gel solutions were loaded into device reservoirs, then one or two droplets were actively dispensed and then manipulated across the patterned hydrophilic sites, where sub-droplets were generated by hydrophobic–hydrophilic interactions [22] . Microgels were formed by incubation for 1–4 h at 37 °C in a humidified chamber or at room temperature, respectively. After formation, individual reagents (for example, fixatives, permeabilizers, dyes and so on, as described below) were delivered to individual microgels by loading the appropriate mixture into a reservoir, actively dispensing a 0.4–2.2 μl droplet onto the array of electrodes, and then passing the droplet across the microgels (passively exchanging the contents of the microgel). UV- and reagent-cross-linked microgel formation Polyacrylamide gels were formed by passive dispensing of an aqueous solution containing 3.6% acrylamide monomer, 0.4% bis-acrylamide cross-linker, 1% w/v VA-086 photo-initiator and 0.05% Pluronics L64. Devices were subsequently filled with either light mineral oil or the fluorinated oil HFE7500 by gentle pipetting at the edge of the top plate, before exposure for 3 min to a UV lamp. After UV exposure, filler oil was removed by applying a kimwipe to the edge of the device top plate. Sodium alginate hydrogels were formed by passive dispensing an aqueous 2% sodium alginate solution followed by engulfing the passively dispensed droplet in a subsequently dispensed droplet of aqueous 2% calcium chloride. Diffusion analysis and modelling Microgels were formed from Geltrex and agarose in 1.5-mm-diameter circular virtual microwells. After 2 h of cross-linking at room temperature in a humidified flask, a droplet of either fluorescein (10 μm in DI water) or fluorescein isothiocyanate-conjugated dextran (4 or 40 kDa, 25 mg ml −1 in DI water) was passed across each hydrogel in a temperature-controlled imaging suite at 23 °C. Each condition was repeated in triplicate. Fluorescent images were recorded at five frames per second (FPS) for up to 3 h. Fifty frames were selected for analysis from each experiment between the onset of diffusion and saturation. Image analysis was performed in ImageJ ( http://rsb.info.nih.gov/ij/ ) by integrating the pixel intensity in a ~1.3-mm-diameter circular region of interest (ROI) within the hydrogelfor each frame over the experimental observation time. The apparent diffusion coefficient ( D a ) was determined by an adaptation of the method reported by Axelrod et al. [57] for fluorescence photobleaching recovery. This model assumes no source density, uniform pore size and no evaporation. Briefly, integrated pixel intensities were normalized to the initial fluorscence intensity of the carrier droplet. These were then plotted with respect to time and the plateau intensity ( A ) was determined. A flourescence saturation half-point ( τ 1/2 ) was defined as the time required for the normalized intensity to reach ½ A . The time constant for diffusion ( τ ) was determined by: An empirical curve was fit to the experimental data: And the apparent diffusion coefficient was set to D a , where r is the radius of the microgel: A numerical simulation was performed using COMSOL Multiphysics ( http://www.comsol.com/ ). A 2D diffusion model was implemented with boundary conditions set to a constant concentration and the respective diffusion coefficients from Equation 3. These experiments were performed with ~150 μm spacers between plates. Composite microgel formation To build composite microgels, a thermally cross-linked microgel was formed initially as described above from either Geltrex or agarose. Secondary hydrogel structures were then formed by manipulating sol-phase hydrogel droplets to surround the initial structures. These were then cross-linked by room temperature incubation and imaged under UV illumination with a digital camera. These experiments were performed with ~150 μm spacers between plates. Before hydrogel seeding sol-phase material was doped with fluorescent latex microspheres to facilitate imaging and gel differentiation. Cell culture MDCK epithelial cells were kindly provided by Dr N. Tufenkji (McGill University). MDCKs were cultured in high-glucose (25 mM) DMEM supplemented with 10% fetal bovine serum (FBS), 100 U ml −1 penicillin and 100 μg ml −1 streptomycin. Microgel cell viability and distribution MDCK cells were prepared at 1 × 10 6 cells per·ml in culture media and then diluted by 50% in 4 °C Geltrex solution. 5 μl aliquots of this suspension were loaded and droplets were actively dispensed across 1.5-mm circular hydrophilic sites to form microgels bearing suspended cells. Each device was then inverted, placed within a Petri dish containing kimwipes saturated with DI water, and incubated at 37 °C in a humidified incubator containing 5% CO 2 for 2 h or 24 h. Cells were then stained by manipulating PBS droplets supplemented with Live/Dead reagents (Life Technologies) and 5 μg ml −1 Hoechst 33342 to exchange the solution with the microgels and then incubated for up to 1 h before exchanging solution with PBS droplets. Cells in the microgels were imaged by confocal microscopy (Zeiss LSM700, Carl Zeiss, Toronto, Canada) at 6-μm increments along the z axis. Viability after cross-linking was determined by enumerating the number of live (green) fluorescent cells and dead (red) fluorescent cells. These experiments were performed with ~225 μm spacers between plates. Epithelialization experiments MDCK cells were seeded in microgels and cultured on devices as described above, but with solution exchange in a fresh droplet of culture medium by passive dispensing every 24 h. Cells on separate devices were fixed at 24, 48, 72, 96 and 120 h after initial seeding by passing three droplets of 10% v/v Histochoice Tissue Fixative in DI water to each hydrogel microgel and then incubating for 30 min at room temperature. Cells were then permeabilized by passing three droplets of permeabilization solution (PS, 0.5% Tween 20 diluted in PBS) across each microgel with 10 min incubation at room temperature between each droplet. Microgels were then labelled with a combination of non-immunological or immunological stains. For the former, Hoechst 33342 was used as above, and Alexa Fluor 488 or 647 phalloidin were delivered by passive dispensing of 5 μg ml −1 solutions in PBS followed by incubation for up to 1 h in the dark. For the latter, label solutions were formed by diluting stock solutions of FITC-conjugated anti-E-cadherin, tight junction protein zonula occludens-1 (ZO-1) mouse monoclonal primary antibody and Alexa Fluor 568 goat anti-mouse secondary antibody in PS 1:50, 1:50 and 1:400, respectively. For E-cadherin and ZO-1 labelling, a droplet of label solution was delivered by passive dispensing followed by incubation for up to 3 h in the dark. For ZO-1 labelling, the microgel was rinsed by delivering three droplets of PS to the microgel by passive dispensing (with 10 min incubation at room temperature after each droplet), followed by delivery of a droplet of secondary antibody label solution by passive dispensing with incubation for up to 3 h in the dark. After all labelling steps, three droplets of PS were passed across each microgel by passive dispensing with 10 min incubation at room temperature between each droplet. Spheroids were then evaluated by bright-field and confocal microscopy (as above), viable spheroids have obvious spheroid shapes and non-viable spheroids appear disorganized and/or blebbed. Cell distribution was determined by recording the z axis position of the largest diameter portion of each individual nucleus in the microgel. Image analysis was performed using Zen Light Edition software (Carl Zeiss, Toronto, Canada). These experiments were performed with ~225 μm spacers between plates. Comparison with conventional fluid handling MDCK spheroids were formed in 3D culture as described above on DMF or in identical reagents in 100 μl gels in 96-well plates. On day 4 of culture, ten randomly selected spheroids for each condition were imaged by light microscopy, followed by reagent exchange. For DMF, this comprised manipulation of five separate 1.2 μl droplets of PBS across the microgel containing spheroids. For 96-well plates, a Biomek FX system (Beckman Coulter, Inc., Fullerton, CA, USA) was used to deliver 100 μl of PBS and then remove 100 μl of PBS at a rate of 50 μl s −1 from each well five times. Spheroids were then re-imaged post manipulation and compared with spheroids pre-manipulation by a measure of circularity using ImageJ to indicate the level of spheroid deformation. Circularity was determined by drawing an ROI along the mid-point of each spheroid (before and after manipulation) and calculated as: Deformation was determined as the absolute per cent change in circularity before and after manipulation, where 100% would indicate complete spheroid disintegration. These experiments were performed with ~225-μm spacers between the plates. Screening experiment Seven devices were each seeded with five 1.5-mm circular microgels containing cells suspended in either Geltrex, Type I collagen or a mixture of the two (1:1 or 3:1 Geltrex:collagen). Geltrex microgels containing MDCK cells were prepared as described above. Collagen microgels were prepared by suspending MDCK cells at 1 × 10 6 cells per·ml in an ice-cold mixture of 0.5 ml collagen Type I (3 mg ml −1 in DMEM with 10% FBS), 62.5 μl 10 × PBS and 62.5 μl of 0.1 M NaOH at pH 7.5 (with pH adjusted with ~10 μl 0.1 N HCl). Aliquots of this suspension (and mixtures of this suspension with appropriate amounts of Geltrex) were loaded, passively dispensed and thermally cross-linked as described above for Geltrex microgels. The devices had inter-plate spacers of 75 or 225 μm, and cells were cultured for 5 days (with media exchange by passive dispensing every 24 h) as above. In some cases, cells were exposed to a droplet of HGF at 20 ng ml −1 in culture media on day 4 and incubated in this solution for the remainder of the experiment. All cells were fixed and stained on-chip as described above on day 5 of culture. A total of 10–15 spheroids were analysed per microgel. Spheroids were evaluated for cross-sectional area and roundness was calculated as: How to cite this article: Eydelnant, I. A. et al. Microgels On-Demand. Nat. Commun. 5:3355 doi: 10.1038/ncomms4355 (2014).